The nuclear hormone receptor PPARγ counteracts vascular calcification by inhibiting Wnt5a signalling in vascular smooth muscle cells Vascular calcification is a hallmark of advanced atherosclerosis. Here we show that deletion of the nuclear receptor PPARγ in vascular smooth muscle cells of low density lipoprotein receptor (LDLr)-deficient mice fed an atherogenic diet high in cholesterol, accelerates vascular calcification with chondrogenic metaplasia within the lesions. Vascular calcification in the absence of PPARγ requires expression of the transmembrane receptor LDLr-related protein-1 in vascular smooth muscle cells. LDLr-related protein-1 promotes a previously unknown Wnt5a-dependent prochondrogenic pathway. We show that PPARγ protects against vascular calcification by inducing the expression of secreted frizzled-related protein-2, which functions as a Wnt5a antagonist. Targeting this signalling pathway may have clinical implications in the context of common complications of atherosclerosis, including coronary artery calcification and valvular sclerosis. Vascular calcification is a frequent complication of atherosclerosis that positively correlates with a high risk of myocardial infarction, hypertension and ischemic episodes in peripheral vascular disease [1] , [2] . In the Framingham Heart Study, patients with cardiovascular disease had a prevalence of vascular calcification of 68% in men and 57% in women at a mean age of 61 years [1] , [3] . Despite its clinical importance, the mechanisms leading to vascular calcifications are not known. Data have converged to indicate that vascular calcification is an actively regulated process similar to the membranous and endochondral bone formation, leading to increased expression of osteogenic and chondrogenic factors, tissue biomineralization and accumulation of cartilage-like cells in the vessel wall [4] . This calcification process is stimulated by bone/vascular morphogens, as well as by autocrine and paracrine Wnt signals [5] , [6] , [7] . The Wnt protein family consists of 22 cysteine-rich secreted glycoproteins, which are involved in many differentiation processes [8] . Inactivation of Wnt-5a in mice or in the chick impairs chondrogenic differentiation and results in abnormal skeletogenesis [9] , [10] . Recently, we reported that the low-density lipoprotein receptor-related protein-1 (LRP1), a multifunctional protein that binds numerous ligands and controls multiple signalling pathways, regulates a canonical Wnt5a signalling pathway in fibroblasts [11] , [12] . LRP1, by inducing the expression of Wnt5a, protects against cholesterol intracellular accumulation [12] . In vivo , LRP1 protects against atherosclerosis [13] . LRP1 negatively controls TGFβ and PDGF signalling [13] , [14] in vascular smooth muscle cells (VSMCs) and disruption of this regulatory mechanism decreases cellular cholesterol export, and leads to foam cell accumulation when mice are fed an atherogenic high-cholesterol diet (Paigen diet) [13] , [14] . Interestingly, treatment of mice in which LRP1 has been selectively ablated in VSMCs (smLRP1−) with rosiglitazone, an agonist of the nuclear receptor PPARγ, normalizes TGFβ signalling and reduces atherosclerotic lesion formation and foam cell accumulation [15] , suggesting a genetic interaction between LRP1 and PPARγ in the vascular wall. PPARγ is involved in a number of differentiation processes. It is a potent activator of adipogenesis [16] and an inhibitor of osteoblast differentiation [17] , [18] . Thus, we hypothesized that LRP1 by stimulating Wnt signalling, and PPARγ by controlling cell differentiation, might jointly control chondrogenesis and vascular calcification. To test this hypothesis, we generated mice that lack PPARγ selectively in VSMCs. We found that these mice, when bred on a low density lipoprotein receptor (LDLr)−/− background to increase atherosclerosis susceptibility, exhibit enhanced Wnt5a expression in the vascular wall and are susceptible to vascular calcification when fed an atherogenic diet. Interestingly, the lack of both PPARγ and LRP1 in VSMCs prevented calcifications. We show that PPARγ counteracts the LRP1/Wnt5a pro-chondrogenic pathway by stimulating the expression of secreted frizzled-related protein-2 (sFRP2). Lack of PPARγ in VSMCs accelerates vascular calcification We generated SM22Cre+/PPARγ flox/flox mice, in which PPARγ is selectively ablated in smooth muscles, by crossing SM22Cre transgenic mice [13] with floxed PPARγ animals (PPARγ flox/flox ) [19] . To increase atherosclerosis susceptibility, SM22Cre+/PPARγ flox/flox animals were maintained on a LDL receptor-deficient background (LDLR−) [20] , and are hereafter referred to as smPPARγ−. Whereas no lesions were seen in smPPARγ− mice fed a regular chow diet, when they were fed an atherogenic diet for 20 weeks, they developed twofold larger atherosclerotic lesions in their aortas than age-matched controls ( Fig. 1a–c ). This is in agreement with a previous report showing that following angiotensin II (angII) perfusion, mice deleted for PPARγ in VSMCs have increased atherosclerosis and aneurysms [21] . Histological analysis of the arterial wall in large vessels such as the aortas and smaller vessels such as the iliac arteries revealed an accumulation of chondrocyte-like cells within the core of the atherosclerotic plaques, whereas reduced macrophage Mac-2-positive and CD-68-positive foam cells accumulated ( Fig. 1d,e ). The atherosclerotic lesion size, as well as the accumulation of chondrocyte-like cells in aortas, was similar in male and female mice ( Fig. 1a,c ; Supplementary Fig. S1a–c ). Von Kossa staining for mineral deposits ( Fig. 1d,e ) showed prominent calcification of the lesions, characteristic of advanced atherosclerosis undergoing vascular mineralization [3] , [22] . In agreement with these results, we found that calcium deposits accumulated in smPPARγ− aortas ( Fig. 1f ). As expected, control mice (smPPARγ+) accumulated Mac2- and CD68-positive foam cells in atherosclerotic plaques ( Fig. 1d ), whereas almost no chondrocyte-like cells were seen ( Supplementary Fig. S1d ). 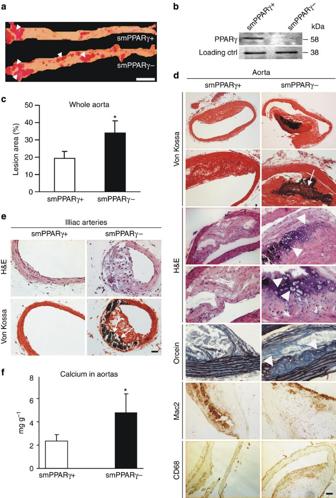Figure 1: Vascular calcification in mice lacking PPARγ in VSMCs and fed a cholesterol-rich diet. (a) Opened and Sudan IV-stained aortas from smPPARγ− male mice and controls (smPPARγ+). Arrowheads show lipid-laden (Sudan-positive) atherosclerotic lesions. Scale bar, 0.5 cm. (b) PPARγ western blotting in aortas. (c) Atherosclerotic lesion size in aortas from smPPARγ− male (n=3) and control (n=4) mice. Error bars, s.d. *P<0.05. (d) Staining of the lesions in aortas. Arrows show calcified lesions and arrowheads show chondrocyte-like cells. Scale bar, VK, 100 μm (top), 50 μm (bottom); Hematoxylin and eosin (H&E), 50 μm (top), 20 μm, (bottom); Orcein (Or), Mac2, and CD68, 20 μm. (e) Staining of the lesions in iliac arteries. Scale bar, 50 μm. (f) Calcium deposits accumulation in aortas from smPPARγ− (n=6) and control (n=7) mice. Error bars, s.e.m. *P<0.05. Figure 1: Vascular calcification in mice lacking PPARγ in VSMCs and fed a cholesterol-rich diet. ( a ) Opened and Sudan IV-stained aortas from smPPARγ− male mice and controls (smPPARγ+). Arrowheads show lipid-laden (Sudan-positive) atherosclerotic lesions. Scale bar, 0.5 cm. ( b ) PPARγ western blotting in aortas. ( c ) Atherosclerotic lesion size in aortas from smPPARγ− male ( n =3) and control ( n =4) mice. Error bars, s.d. * P <0.05. ( d ) Staining of the lesions in aortas. Arrows show calcified lesions and arrowheads show chondrocyte-like cells. Scale bar, VK, 100 μm (top), 50 μm (bottom); Hematoxylin and eosin (H&E), 50 μm (top), 20 μm, (bottom); Orcein (Or), Mac2, and CD68, 20 μm. ( e ) Staining of the lesions in iliac arteries. Scale bar, 50 μm. ( f ) Calcium deposits accumulation in aortas from smPPARγ− ( n =6) and control ( n =7) mice. Error bars, s.e.m. * P <0.05. Full size image mRNA levels encoding chondro-osteogenic proteins, such as the Fos-related AP1 transcription factor Fra2 [5] , Col10a1, osteocalcin, alkaline phosphatase (ALP), Runx2 and Col2a, which promote mineralization [23] , were significantly increased in aortas of male and female smPPARγ− mice ( Fig. 2a ; Supplementary Fig. S1e ). Moreover, high transcript levels of the transcription factor sex-determining region Y (SRY)-box 9 (Sox9), a master regulator of chondrogenesis [24] , and of the transcription factor cartilage homeoprotein 1 (Cart1) [7] , which has been reported to stimulate chondrogenesis in bone and in the vascular wall [5] , [6] , [7] were found in the core of the lesions ( Fig. 2b ). To test whether PPARγ−/− VSMCs can differentiate into chondrocyte-like cells in vitro , VSMCs isolated from aortas of 3- to 4-month-old smPPARγ− mice were treated with a chondrogenic cocktail for 15 days. Alizarin red and Alcian blue staining revealed that VSMCs PPARγ−/− accumulated mineral deposits ( Fig. 2c ). Transcript levels of the chondrogenic markers Sox9 and Cart 1 were increased compared with controls ( Fig. 2d ). Similar results were obtained in primary cultured PPARγ−/− skin fibroblasts treated with a chondrogenic cocktail ( Supplementary Fig. S2a,b ). Thus, the expression of PPARγ in VSMCs inhibits the expression of chondrogenic and osteogenic markers, and protects against the accumulation of chondrocyte-like cells in the arterial wall. Interestingly, mRNA levels of the vascular smooth muscle cell markers myosin heavy chain (SMMHC) and smooth muscle Actin (sm-Actin) were reduced in aortas from SM22Cre+/PPARγ flox/flox LDLr−/− (smPPARγ−) mice ( Fig. 2e ), suggesting that PPARγ-deficient cells had partly lost their smooth muscle phenotype, and had differentiated towards a chondrocytic lineage. 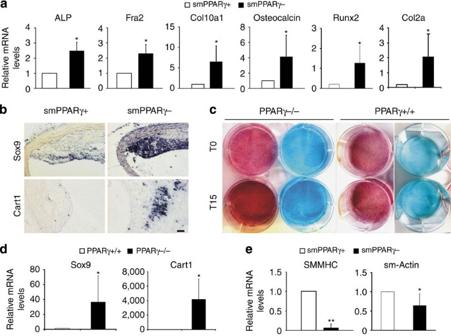Figure 2: Expression of functional markers in aortas from smPPARγ− mice. (a) RT–PCR analysis and (b)in situhybridization of the indicated genes in aortas from smPPARγ− (n=5) and control mice (n=5) fed an atherogenic diet. Scale bar, 50 μm. (c) Alizarin red (left panels of each genotype) and alcian blue (right panels of each genotype) staining of VSMCs isolated from smPPARγ− and control mice aortas and treated (T15) or not (T0) with a chondrogenic cocktail for 15 days. (d) RT–PCR analysis of the indicated genes of VSMCs isolated from smPPARγ mice aortas treated 15 days for chondrogenesis (each genotypen=5). (e) RT–PCR analysis of VSMC-selective markers in aortas from smPPARγ− mice (n=5) and controls (n=5). Error bars, s.d. *P<0.05; **P<0.01. Figure 2: Expression of functional markers in aortas from smPPARγ− mice. ( a ) RT–PCR analysis and ( b ) in situ hybridization of the indicated genes in aortas from smPPARγ− ( n =5) and control mice ( n =5) fed an atherogenic diet. Scale bar, 50 μm. ( c ) Alizarin red (left panels of each genotype) and alcian blue (right panels of each genotype) staining of VSMCs isolated from smPPARγ− and control mice aortas and treated (T15) or not (T0) with a chondrogenic cocktail for 15 days. ( d ) RT–PCR analysis of the indicated genes of VSMCs isolated from smPPARγ mice aortas treated 15 days for chondrogenesis (each genotype n =5). ( e ) RT–PCR analysis of VSMC-selective markers in aortas from smPPARγ− mice ( n =5) and controls ( n =5). Error bars, s.d. * P <0.05; ** P <0.01. Full size image Molecular mechanisms leading to increased calcification As Wnt5a has been shown to initiate differentiation of chondrocytes in vitro and in vivo [25] , we tested whether it might also be involved in the phenotype observed in smPPARγ− mice. Wnt5a transcripts levels in aortas from these mice were twofold increased compared with controls ( Fig. 3a ). Interestingly, we found an intense Wnt5a immunoreactivity in atherosclerotic lesions from human carotid arteries ( Fig. 3b ) and a marked increase in Wnt5a mRNA levels ( Fig. 3c ) in calcified regions. To determine whether Wnt5a can activate the chondrogenic program, we used LRP1−/− mouse embryonic fibroblasts (MEFs) that do not express endogenous Wnt5a [12] . We show that recombinant Wnt5a strongly stimulates luciferase expression driven by the Cart1 and Sox9 promoters ( Fig. 3d ; Supplementary Fig. S2c ). Thus, Wnt5a can activate essential components of the chondrogenic program, and its increased expression in arteries is associated with chondrogenic metaplasia in mice, as well as in humans. 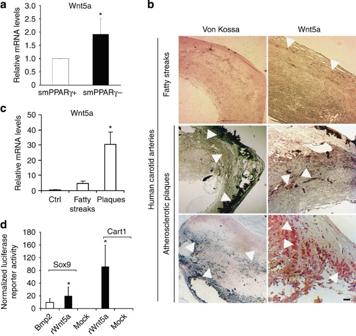Figure 3: Wnt5a expression correlates with calcification in mice and human arteries. (a) Wnt5a mRNA levels in aortas from smPPARγ− (n=5) and control mice (n=5) fed an atherogenic diet. (b) Immunohistochemistry and Von Kossa staining, and (c) RT–PCR analysis of Wnt5a in atherosclerotic lesions from human internal mammary (Ctrl,n=3), and human carotid arteries with (atherosclerotic plaques) and without (fatty streaks) calcified lesions (n=4). Arrowheads show Wnt5a labeling (in red) and calcified lesions. Scale bar, 50 μm. (d) Luciferase reporter activity in LRP1−/− MEFs transiently transfected with luciferase reporter containing theSox9or theCart1promoter, and treated with 100 ng ml−1purified recombinant Wnt5a, mock fraction (without Wnt5a) or BMP2 as positive control (100 ng ml−1) (n=4). Error bars, s.d. *P<0.05. Figure 3: Wnt5a expression correlates with calcification in mice and human arteries. ( a ) Wnt5a mRNA levels in aortas from smPPARγ− ( n =5) and control mice ( n =5) fed an atherogenic diet. ( b ) Immunohistochemistry and Von Kossa staining, and ( c ) RT–PCR analysis of Wnt5a in atherosclerotic lesions from human internal mammary (Ctrl, n =3), and human carotid arteries with (atherosclerotic plaques) and without (fatty streaks) calcified lesions ( n =4). Arrowheads show Wnt5a labeling (in red) and calcified lesions. Scale bar, 50 μm. ( d ) Luciferase reporter activity in LRP1−/− MEFs transiently transfected with luciferase reporter containing the Sox9 or the Cart1 promoter, and treated with 100 ng ml −1 purified recombinant Wnt5a, mock fraction (without Wnt5a) or BMP2 as positive control (100 ng ml −1 ) ( n =4). Error bars, s.d. * P <0.05. Full size image As recent genetic experiments have shown that sFRP2, a Wnt antagonist member of the sFRP family, is a potent inhibitor of chondrogenesis [26] , we tested whether PPARγ stimulates the expression of sFRP2 in VSMCs. sFRP2 transcripts were reduced to almost undetectable levels in aortas from smPPARγ− mice ( Fig. 4a ), whereas transcripts of other sFRPs such as sFRP1 remained unchanged ( Supplementary Fig. S2d ), suggesting that sFRP2 is a PPARγ target gene. We also found a putative PPARγ response element (PPRE) [27] , [28] located between nucleotides −897 and −884 of the sFRP2 promoter ( Supplementary Fig. S3a ). Chromatin immunoprecipitation experiments showed that PPARγ binds to the sFRP2 promoter region encompassing this PPRE in MEFs treated with an adipogenic cocktail containing rosiglitazone to induce PPARγ expression and activity ( Fig. 4b ). These data demonstrate that PPARγ controls expression of the Wnt antagonist sFRP2 at the transcriptional level. To test whether sFRP2 can inhibit the chondrogenic program in VSMCs, we treated wild-type human VSMCs (HUVSMCs) for 24 h with recombinant sFRP2 or with the PPARγ agonist rosiglitazone. Both treatments decreased Cart1 mRNA levels ( Fig. 4c ). Treatment for 15 days of PPARγ−/− VSMCs isolated from aortas of smPPARγ− mice with a chondrogenic cocktail containing recombinant sFRP2 greatly decreased Sox9 and Cart1 mRNA levels ( Fig. 4d,e ) and inhibited mineralization ( Fig. 4f ). However, treatment of these cells for 15 days with 10 μM rosiglitazone did not inhibit chondrogenesis ( Fig. 4g ). Similarly, treatment of smPPARγ− mice with rosiglitazone for 2 months did not reduce vascular calcification ( Fig. 4h , Supplementary Fig. S2e,f ). Thus, PPARγ by positively controlling sFRP2 expression inhibits chondrogenesis in VSMCs. 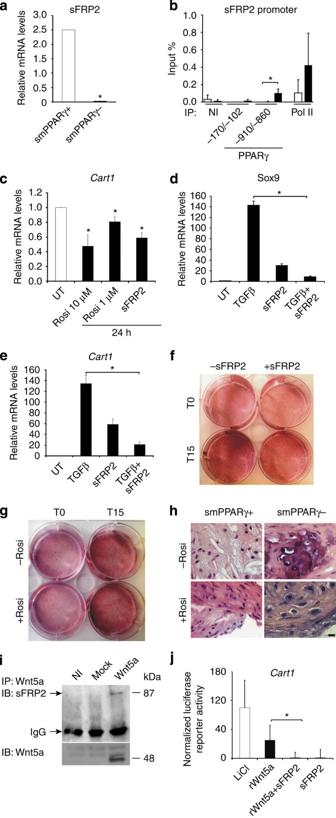Figure 4: sFRP2 inhibits chondroid metaplasia in aortas and VSMCs. (a) sFRP2 mRNA levels in aortas from smPPARγ− (n=5) and control mice (n=5) fed an atherogenic diet. (b) ChIP analysis of PPARγ binding to the sFRP2 promoter region containing (−910/−860) or not (−170/−102) PPREs (n=3). (c) mRNA levels of Cart1 in wild-type human VSMCs treated for 24 h with a chondrogenic cocktail containing 1–10 μM rosiglitazone, or recombinant sFRP2 (300 ng ml−1). (d) Sox9 and (e) Cart1 mRNA levels in VSMCs from aortas of smPPARγ− mice treated for 15 days with a chondrogenic cocktail containing or not (UT) sFRP2 (300 ng ml−1). (f) Alizarin red staining of VSMCs isolated from PPARγ−/− aortas and treated for chondrogenesis +/− recombinant sFRP2 during 15 days. (g) Alizarin red staining of VSMCs isolated from aortas of smPPARγ− mice and treated for 15 days with a chondrogenic cocktail containing (T15) or not (T0) 1 μM rosiglitazone. (h) Histological analysis and Hematoxylin and eosin (H&E) staining of aortas from smPPARγ− and control mice fed an atherogenic diet + rosiglitazone. Scale bar, 20 μm. (i) Co-immunoprecipitation between Wnt5a and endogenous sFRP2 in HEK 293 cells transiently transfected with a Wnt5a-myc construct. NI, non-immune. IB, immunoblot; IP, immunoprecipitation. (j) Luciferase reporter activity in LRP1−/− MEFs transiently transfected with luciferase reporter containing theCart1promoter, and treated with 100 ng ml−1purified recombinant Wnt5a (rWnt5a), recombinant sFRP2 (300 ng ml−1) or LiCl as positive control (50 mM) (n=3). Error bars, s.d. *P<0.05. Figure 4: sFRP2 inhibits chondroid metaplasia in aortas and VSMCs. ( a ) sFRP2 mRNA levels in aortas from smPPARγ− ( n =5) and control mice ( n =5) fed an atherogenic diet. ( b ) ChIP analysis of PPARγ binding to the sFRP2 promoter region containing (−910/−860) or not (−170/−102) PPREs ( n =3). ( c ) mRNA levels of Cart1 in wild-type human VSMCs treated for 24 h with a chondrogenic cocktail containing 1–10 μM rosiglitazone, or recombinant sFRP2 (300 ng ml −1 ). ( d ) Sox9 and ( e ) Cart1 mRNA levels in VSMCs from aortas of smPPARγ− mice treated for 15 days with a chondrogenic cocktail containing or not (UT) sFRP2 (300 ng ml −1 ). ( f ) Alizarin red staining of VSMCs isolated from PPARγ−/− aortas and treated for chondrogenesis +/− recombinant sFRP2 during 15 days. ( g ) Alizarin red staining of VSMCs isolated from aortas of smPPARγ− mice and treated for 15 days with a chondrogenic cocktail containing (T15) or not (T0) 1 μM rosiglitazone. ( h ) Histological analysis and Hematoxylin and eosin (H&E) staining of aortas from smPPARγ− and control mice fed an atherogenic diet + rosiglitazone. Scale bar, 20 μm. ( i ) Co-immunoprecipitation between Wnt5a and endogenous sFRP2 in HEK 293 cells transiently transfected with a Wnt5a-myc construct. NI, non-immune. IB, immunoblot; IP, immunoprecipitation. ( j ) Luciferase reporter activity in LRP1−/− MEFs transiently transfected with luciferase reporter containing the Cart1 promoter, and treated with 100 ng ml −1 purified recombinant Wnt5a (rWnt5a), recombinant sFRP2 (300 ng ml −1 ) or LiCl as positive control (50 mM) ( n =3). Error bars, s.d. * P <0.05. Full size image To test whether sFRP2 is a Wnt5a antagonist, an expression vector encoding a Wnt5a-myc tagged protein was transfected into Human Embryonic Kidney HEK 293 cells that express high sFRP2 levels. Immunoprecipitation of the Wnt5a-myc protein from the extracellular medium using anti-myc antibodies revealed a physical interaction between sFRP2 and Wnt5a ( Fig. 4i ). Moreover, recombinant sFRP2 strongly antagonized Wnt5a-induced activation of the Cart1 promoter in LRP1−/− MEFs ( Fig. 4j ). Taken together, these data strongly suggest that PPARγ prevents vascular calcification by stimulating the expression of sFRP2, an antagonist of the Wnt5a prochondrogenic pathway. LRP1 in VSMCs is required for vascular calcification We previously reported that LDLr−/− mice lacking LRP1 in VSMCs (smLRP1−) develop atherosclerotic lesions [13] with accumulation of foam cells in their vascular wall [29] . Interestingly, no vascular calcification was described in these mice, suggesting that LRP1 might be required for vascular calcification. To test this, we measured the expression of chondrogenic markers in aortas from smLRP1− mice and found that Sox9 and Cart1 ( Fig. 5a ), as well as ALP mRNA levels ( Supplementary Fig. S3b ) were unchanged compared with controls. Atherosclerotic lesions in smLRP1− mice consisted mainly of macrophage Mac-2-positive and CD68-positive foam cell accumulation, and Von Kossa staining confirmed the absence of calcification ( Fig. 5a ). We also found low mRNA levels of Wnt5a in aortas from smLRP1− mice ( Fig. 5b ), whereas sFRP2 mRNA levels remained unchanged compared with controls ( Supplementary Fig. S3c ). Moreover, in vitro , primary cultured LRP1−/− VSMCs, as well as skin fibroblasts, were resistant to differentiation when treated with a chondrogenic cocktail for 15 days ( Fig. 5c and Supplementary Fig. S3d ). mRNA levels of Cart1 and Sox9 were much less induced than in LRP1+/+ cells ( Fig. 5d ; Supplementary Fig. S3e ). 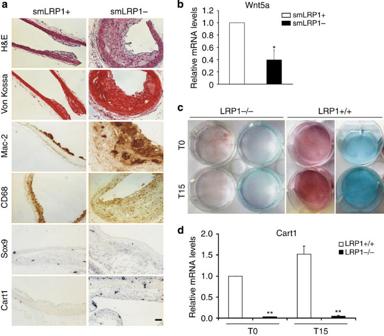Figure 5: LRP1 is required for chondroid metaplasia in aortas. (a) Histological analysis and Hematoxylin and eosin (H&E) staining, Von Kossa staining, immunostaining with Mac-2 and CD68 antibodies, andin situhybridization with Sox9 and Cart1 antisense probes in opened aortas from smLRP1− mice fed a cholesterol-rich diet. Scale bar, 50 μm. (b) Wnt5a mRNA levels in aortas from smLRP1− (n=5) and control mice (n=5). (c) Alizarin red (left panels of each genotype) and alcian blue (right panels of each genotype) staining, and (d) Cart1 mRNA levels in VSMCs isolated from aortas of smLRP1− mice and treated with a chondrogenic cocktail for 15 days (n=4). Error bars, s.d. *P<0.05; **P<0.01. Figure 5: LRP1 is required for chondroid metaplasia in aortas. ( a ) Histological analysis and Hematoxylin and eosin (H&E) staining, Von Kossa staining, immunostaining with Mac-2 and CD68 antibodies, and in situ hybridization with Sox9 and Cart1 antisense probes in opened aortas from smLRP1− mice fed a cholesterol-rich diet. Scale bar, 50 μm. ( b ) Wnt5a mRNA levels in aortas from smLRP1− ( n =5) and control mice ( n =5). ( c ) Alizarin red (left panels of each genotype) and alcian blue (right panels of each genotype) staining, and ( d ) Cart1 mRNA levels in VSMCs isolated from aortas of smLRP1− mice and treated with a chondrogenic cocktail for 15 days ( n =4). Error bars, s.d. * P <0.05; ** P <0.01. Full size image To further demonstrate that LRP1 is required for vascular calcification, we generated LDLr−/− mutant mice in which both PPARγ and LRP1 were selectively ablated in VSMCs (smPPARγ−/smLRP1−) and fed them an atherogenic diet for 20 weeks. In these mice, the area covered by atheromas ( Fig. 6a ), as well as the accumulation of macrophage Mac-2-positive and CD68-positive foam cells ( Fig. 6b ), were similar to that of smLRP1− mice. No accumulation of chondrocytes or calcium deposits was seen in the aortas of these mice ( Fig. 6b,c ). mRNA levels of Sox9, Cart1 ( Fig. 6b ), ALP ( Supplementary Fig. S3f ), as well as Wnt5a ( Fig. 6e ) remained unchanged, whereas sFRP2 mRNA levels were reduced ( Fig. 6d ). When treated with a chondrogenic cocktail for 15 days VSMCs isolated from aortas of smLRP1−/smPPARγ− mice were resistant to differentiation ( Supplementary Fig. S3g ). mRNA levels of Cart1 and Sox9 remained unchanged in these cells ( Supplementary Fig. S3h ). Thus, LRP1 in VSMCs is required for vascular calcification by promoting a prochondrogenic Wnt5a signalling, which is antagonized by the PPARγ target gene, sFRP2 ( Fig. 7 ). 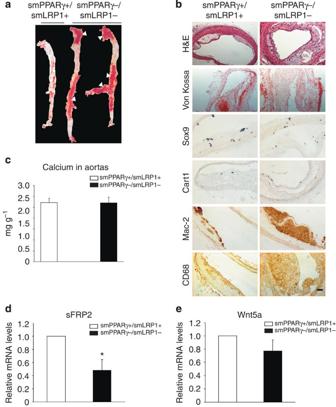Figure 6: smLRP1−/smPPARγ− mice are protected against vascular calcification. (a) En-face analysis of Sudan IV-stained aortas from smPPARγ−/smLRP1− mice that have been fed a cholesterol-rich diet for 20 weeks. (b) Hematoxylin and eosin (H&E), Von Kossa staining, immunostaining with Mac-2 and CD68 antibodies andin situhybridization with Sox9 and Cart1 antisense probes in opened aortas from smLRP1−/smPPARγ− mice fed a cholesterol-rich diet. Scale bars, 50 μm. (c) Calcium deposits accumulation in aortas from smPPARγ−/smLRP1− (n=5) and control (n=4) mice. (d) sFRP2 and (e) Wnt5a mRNA levels in aortas from smLRP1−/smPPARγ− (n=5) and control mice (n=5). Error bars, s.d. *P<0.05. Figure 6: smLRP1−/smPPARγ− mice are protected against vascular calcification. ( a ) En-face analysis of Sudan IV-stained aortas from smPPARγ−/smLRP1− mice that have been fed a cholesterol-rich diet for 20 weeks. ( b ) Hematoxylin and eosin (H&E), Von Kossa staining, immunostaining with Mac-2 and CD68 antibodies and in situ hybridization with Sox9 and Cart1 antisense probes in opened aortas from smLRP1−/smPPARγ− mice fed a cholesterol-rich diet. Scale bars, 50 μm. ( c ) Calcium deposits accumulation in aortas from smPPARγ−/smLRP1− ( n =5) and control ( n =4) mice. ( d ) sFRP2 and ( e ) Wnt5a mRNA levels in aortas from smLRP1−/smPPARγ− ( n =5) and control mice ( n =5). Error bars, s.d. * P <0.05. 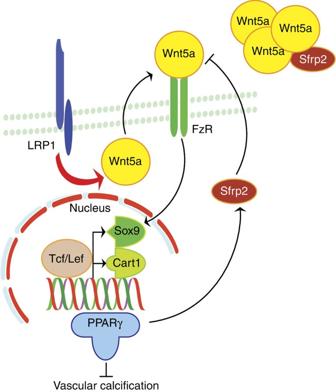Figure 7: A schematic diagram of LRP1-dependent vascular calcification. When mice are fed an atherogenic diet, vascular calcification is induced if LRP1 is expressed in VSMCs. LRP1 positively regulates a Wnt5a signalling pathway that activates chondrogenic-specific genes in the vascular wall. PPARγ and its target sFRP2 protect against vascular calcification by inhibiting the pro-chondrogenic Wnt5 pathway. Conversely, in the absence of LRP1, Wnt5a signaling is inhibited, which promotes intracellular cholesterol accumulation and foam cell development. Full size image Figure 7: A schematic diagram of LRP1-dependent vascular calcification. When mice are fed an atherogenic diet, vascular calcification is induced if LRP1 is expressed in VSMCs. LRP1 positively regulates a Wnt5a signalling pathway that activates chondrogenic-specific genes in the vascular wall. PPARγ and its target sFRP2 protect against vascular calcification by inhibiting the pro-chondrogenic Wnt5 pathway. Conversely, in the absence of LRP1, Wnt5a signaling is inhibited, which promotes intracellular cholesterol accumulation and foam cell development. Full size image The mechanisms underlying vascular calcification have been difficult to study because of the lack of appropriate animal models. Previous studies suggested that PPARγ [30] , [31] is involved in ectopic calcification, but the underlying molecular mechanism was unclear. In the present study, we identified a functional interaction between PPARγ and LRP1 in VSMCs of mice that leads to calcified lesions of arteries resembling those seen in humans. We show that mice fed a high-cholesterol diet develop enhanced vascular calcification when PPARγ is selectively deleted in VSMCs ( Fig. 1e,f ). Proteins inducing osteoblastic and chondrocytic differentiation, such as Sox9, ALP, Cart1 and osteocalcin, were upregulated in calcified atherosclerotic lesions of smPPARγ-deficient vessels. We have shown that the levels of the Wnt inhibitor sFRP2 are strongly reduced in vessels of smPPARγ− mice, allowing activation of Wnt5a signalling, which promotes calcification of mice. In addition, we show that Wnt5a levels are overexpressed in human atherosclerotic lesions undergoing calcification. We also provide evidence that PPARγ binds to the sFRP2 promoter and stimulates sFRP2 expression. Recent experiments have shown that sFRP2 inhibits both osteogenic and chondrogenic lineage commitment of mesenchymal stem cells [32] , and that its overexpression decreases calcification within infarcted myocardium [32] . Here we show that sFRP2 inhibits chondrogenesis of PPARγ−/− VSMCs. In wild-type VSMCs, a treatment with the PPARγ ligand rosiglitazone or with recombinant sFRP2 decreases the expression of chondrogenic markers. Conversely, sFRP2 inhibits chondrogenesis of PPARγ-deficient VSMCs and rosiglitazone does not inhibit chondrogenesis in PPARγ−/− VSMCs, as well as in smPPARγ− mice. Thus, by inducing the expression of sFPR2, PPARγ protects against vascular calcification. sFRP2 is a secreted protein that has been described to antagonize Wnt1 and Wnt9a [26] . Here we show that it also interacts with Wnt5a [9] , [10] , a regulator of chondrogenesis. sFRP2 is expressed in proliferating and prehypertrophic chondrocytes [33] . Its ablation in mice leads to abnormal skeletogenesis, whereas overexpression is associated with a delay in chondrocyte maturation [34] . The mechanism by which Wnt5a regulates the chondrogenic program was unknown. In the present study, we have shown that Wnt5a induces the expression of two regulators of chondrogenesis, Sox9 and Cart1, and this is associated with ectopic chondrogenesis in the vessel wall. Moreover, we have demonstrated that mice selectively lacking LRP1 or both LRP1 and PPARγ in VSMCs and fed an atherogenic diet, exhibit low levels of Wnt5a in the aorta, and are protected against vascular calcifications. Taken together, these data demonstrate that the expression of LRP1 in VSMCs is required for vascular calcification to occur, and that PPARγ by counteracting the LRP1/Wnt5a pro-chondrogenic pathway protects against vascular calcification. PPARγ is known to act as a transcriptional sensor that translates stimuli from the local environment into adaptive metabolic responses. For instance, PPARγ is essential for adipogenesis, which is induced by lipogenic stimuli [35] , but it is also a key repressor of osteoblastogenesis [36] , [37] . In vitro data suggest that PPARγ activation stimulates adipocyte differentiation of mesenchymal stromal precursor cells at the expense of osteoblastogenesis. A similar switch may occur in vivo in VSMCs, where in the absence of PPARγ, VSMCs undergo a phenotypic change towards the chondrocytic lineage [38] . This process is affected by the composition of the diet, as it occurs only in mice fed an atherogenic high-cholesterol diet. The notion that VSMCs can undergo phenotypic changes has been previously reported [39] . Indeed, VSMCs can give rise to chondrocytes [40] and have important roles in the initiation and progression of vascular calcification [40] , [41] . Moreover, it has previously been suggested that arterial calcification is associated with a decrease in smooth muscle lineage markers, and an increase in chondrogenic markers [42] . Here, we report a decrease in the mRNA levels of the VSMCs markers MHC and sm-Actin in aortas from smPPARγ− mice, indicating that cells have partly lost their characteristic contractile phenotype [43] , an event that may facilitate their differentiation toward the chondrocytic lineage. Alternatively, albeit unlikely, chondrocyte-like cells that accumulate in the media of blood vessels from smPPARγ− mice originate from monocyte-macrophages that have lost Mac-2 and CD68 expression. In summary, our data show that LRP1 and PPARγ are important determinants for chondrocyte differentiation in the vascular wall and for vascular calcification induced during atherosclerosis. By positively regulating a canonical Wnt5a signalling pathway, LRP1 is a pro-chondrogenic factor in the vascular wall. PPARγ, in contrast, by enhancing the expression of the Wnt5a inhibitor sFRP2, counteracts the LRP1-mediated chondrogenic program ( Fig. 7 ), and acts as an inhibitor of vascular calcification. Our findings may have important clinical implications, as they indicate that selective PPARγ agonists such as thiazolidinediones might have therapeutic value for the treatment and prevention of artery calcifications. Animals The generation of LDLR knockout, LRP1 flox/flox SM22Cre and PPARγ flox/flox animals has been reported earlier [13] , [19] . Mice in which LRP1 was ablated in VSMC are referred to as smLRP1− (SM22Cre+; LRP1 flox/flox LDLr−/−), and their littermate controls are referred to as smLRP1+ (LRP1 flox/flox ;LDLr−/−). Mice in which PPARγ was ablated in VSMC are referred to as smPPARγ− (SM22Cre+; PPARγ flox/flox LDLr−/−), and their littermate controls are referred to as smPPARγ+ (PPARγ flox/flox ;LDLr−/−). Animals were maintained on a 12-h light/12-h dark cycle. As most of the smLRP1− mice and the smLRP1/smPPARγ double mutants died when fed a Paigen diet for more than 11 (ref. 13 ) or 20 weeks, respectively, mice were fed a standard laboratory chow (UAR, Villemoison sur Orge, France) or a Paigen diet for a maximum of 11 weeks for the smLRP1, and 20 weeks for the smPPARγ mice and the smLRP1/smPPARγ double mutants. All animals used in the experiments were age- and sex-matched and littermates. Experiments were conducted according to procedures approved by the Institutional Animal Care and Use Committee at University of Strasbourg, France. For histological analysis, mice were transcardially perfused with a 4% paraformaldehyde solution in phosphate-buffered saline. Entire aortas were dissected, opened and stained with Sudan IV to reveal lipid-filled atherosclerotic lesions [13] . Hematoxylin/Eosin and Von Kossa staining were performed according to standard methods. For calcium measurement, aortic samples were weighted, dried at 105 °C, and mineralized in concentrated HNO 3 . The solution was filtered (0.45 μm) and the volume adjusted to 20 ml with H 2 O. Solution was analysed by inductively coupled Plasma Optical Emission Spectrometers at 396.8 nm. For rosiglitazone treatments, rosiglitazone maleate was mixed into the paigen diet at 25 mg kg −1 per day for 2 months. Human samples Human carotid endarterectomy samples containing calcified atherosclerotic lesions were obtained from the Vascular Surgery Department (Groupe Hospitalier Pitié-Salpétrière, Paris). Fragments of left internal mammary arteries, remaining after coronary artery bypass graft surgery, were obtained from the Cardiovascular Department (Centre Hospitalier Intercommunal, Créteil). An informed consent from all patients was obtained. For Von Kossa staining, sections were de-paraffinized and hydrated to water. Sections were incubated with 1% silver nitrate solution in the darkness for 30 min. After rinsing with distilled water, un-reacted silver was removed with 5% sodium thiosulfate for 5 min. Slides were then counterstained with nuclear fast red for 5 min. In situ hybridization Mouse aortas were embedded in OCT (Tissue-Tek; Miles) and frozen in dry ice. Sections (10 μm) were thaw mounted onto slides (Superfrost plus, Menzel-Glaser) and stored at −80 °C. Complementary DNA (cDNA) fragments for mouse Sox9, Cart1 and VEGFr were subcloned to synthesize antisense probes. Digoxigenin-11-UTP RNA sense and antisense riboprobes were transcribed in the presence of UTP-11-Digoxigenin by T7 and T3 RNA polymerases. After probe hybridization, slides were coated with anti-digoxigenin antibody conjugated with Alkaline phosphatase and stained in NTMT (NaCl 100 mM, Tris 100 mM pH 9.5, MgCl 2 /6H 2 O 50 mM, Tween-20 0.1%), NBT (nitroblue tetrazolium)/BCIP (5-bromo-4-chloro-3-indolyl-phosphate) buffer. Cell culture and immunoprecipitation experiments Cells were seeded in 100 mm dishes and grown to 80% confluence in Dulbecco's modified Eagle's medium (DMEM) (Invitrogen, CA) supplemented with 10% (v/v) new-born calf serum. Adipocyte differentiation was induced as described [12] . For primary cultured VSMCs and skin fibroblasts, thoracic aortas and skin from 8-week-old male smLRP1−, smPPARγ−, smLRP1−/smPPARγ− and controls mice were dissected free from connective tissue. After 15 min at 37 °C in DMEM supplemented with NSC 10% and collagenase 0.1%, the aortas were opened longitudinally and the intima scraped on luminal surface. Tissue samples were minced into small pieces and placed into a T25 flask with high-glucose (4.5 g l −1 ) DMEM containing 15% fetal bovine serum, 100 U ml −1 penicillin, 100 mg ml −1 streptomycin, 20 mM L -glutamine. Both explants and cells were cultured at 37 °C in 5% carbon dioxide (CO 2 ). Cells were detached by incubation with 0.25% trypsin-EDTA solution. Passages 4–7 were used in this study. Chondrogenic differentiation was induced with TGFβ (10 ng ml −1 ) for 15 days in 10% FCS/DMEM. Immunoprecipitation experiments were done as described previously [13] . Briefly, cells were washed with ice-cold PBS and lysed for 20 min on ice in lysis buffer supplemented with protease inhibitors. The lysates were precleared, then incubated overnight at 4 °C with the indicated antibody and protein A-Sepharose CL-4B beads. Immunoprecipitates were washed twice with lysis buffer and lysis buffer containing 2 M NaCl, and twice in 10 mM Tris, pH 8, 50 mM NaCl. Proteins were eluted from beads with SDS sample buffer, separated by SDS–polyacrylamide gel electrophoresis, transferred to nitrocellulose membrane and blotted with the indicated antibody. Recombinant proteins Purification of the murine recombinant Wnt5a was described earlier [44] . Cells were infected with 100 ng ml −1 purified recombinant Wnt5a. Infected cell supernatant was cleared by centrifugation at 4 °C, aliquoted and stored at −20 °C until use. The Myc-tagged Wnt5a construct [12] was clone into the pcDNA 3.1 Zeo (Invitrogen). Gene expression analysis RNA was isolated using TRIzol reagent (Sigma, St Louis) according to the manufacturer's instructions. A total of 50 ng of RNA was converted to cDNA using the high-capacity cDNA Archive kit (Applied Biosystems, Foster City, CA). PCR amplification was performed using SYBRGreen PCR master mix (Applied Biosystems) according to the manufacturer's instructions. Primers sequences are: ALP: forward (for.) 5′-CCTGAAACTCCCAAAAGCTC-3′, reverse (rev.) 5′-TCTGGTGGCATCTCGTTATC-3′; Fra2: for. 5′-GAGTGATCAAGACCATCGGTACC-3′, rev. 5′-AGACAGCTGCTCATCTCTCCTTC-3′; Col10a1: for. 5′-CTTTGTGTGCCTTTCAATCG-3′, rev. 5′-GTGAGGTACAGCCTACCAGTTTT-3′; Osteocalcin: for. 5′-CTCTGTCTCTCTGACCTCACAG-3′, rev. 5′-GGAGCTGCTGTGACATCCATAC-3′; Runx2: for. 5′-GAGGGCACAAGTTCTATCTGGA-3′, rev. 5′-GGTGGTCCGCGATGATCTTC-3′; Col2a: for. 5′-ACACTGGGAATGTCCTCTGC-3′, rev. 5′-ACCTGCCAGACCATCTTGAC-3′; Sox9: for. 5′-AGCAAGAACAAGCCACACGTC-3′, rev. 5′-TCGTTCAGCAGCCTCCAGA-3′; Cart1: for. 5′-CAATGGATAACTGCAACAATCTCAG-3′, rev. 5′-CTGGATACATTGCTGTCACATTTG-3′; SMMHC: for. 5′-CACCTGGAGAGGATGAAGAAGAA-3′, rev. 5′-AAGACTTGACTTTCACTTGGAGTTTATC-3′; SmActin: for. 5′-ATCGTCCACCGCCAAATGC-3′, rev. 5′-AAGGAACTGGAGGCGCTG-3′; Wnt5a: for. 5′-GCAGACCGAACGCTGTCAT-3′, rev. 5′-CCTTCACCTGGATACCACCCA-3′; Sfrp2: for. 5′-ACGACAACGACATCATGGAA-3′, rev. 5′-ACGCCGTTCAGCTTGTAAAT-3′; Sfrp1: for. 5′-GCCACAACGTGGGCTACAA-3′, rev. 5′-ACCTCTGCCATGGTCTCGT-3′; GAPDH: for. 5′-TGTGTCCGTCGTGGATCTGA-3′, rev. 5′-CCTGCTTCACCACCTTCTTGAT-3′. Reporter gene assay The Sox9 (−2 kb) [45] and the Cart1 promoter ( Supplementary Fig. S2b ) linked to a luciferase reporter were transiently transfected in HEK 293 cells or MEFs using a calcium phosphate standard method. At 48 h after the transfection, cells were collected and reporter gene assays were carried out using the Luciferase assay system (Promega). Transfection efficiency was normalized by measuring expression of β-galactosidase activity and background activity was subtracted. Mock is the luciferase activity in the absence of exogenous Wnt5a. Antibodies and immunoblotting SDS–polyacrylamide gel electrophoresis and immunoblot analysis were performed according to standard procedures. Proteins were transferred onto nitrocellulose membranes and immunoblot analyses were carried out using antibodies directed against β-catenin (1/1,000), sFRP2 (1/1,000), LRP1 (1/1,000), c-Myc (1/500) (R&D systems, Minneapolis, MN), or GAPDH (1/10,000) (Sigma). Chromatin immunoprecipitation ChIPs were performed on MEF cells for three or more biological replicates as described [46] . Non-specific controls were performed with samples incubated with sepharose beads in the presence of non-immune antibodies. Primer sequences were designed to amplify the specific 5′-897-GAGGTCAAATTTCTCCTC–881-3′ promoter region of sFRP2. Results are expressed relative to the amount of input DNA per ChIP. Statistical analysis Values are reported as mean±s.d. of at least triplicate determinations. For in vivo analysis, 3–6 male and female mice were used for each genotype. Statistical significance ( P <0.05) was determined by unpaired Student's t -test (Statview, Abacus Concepts, Berkeley, CA). How to cite this article: Woldt, E. et al . The nuclear hormone receptor PPARγ counteracts vascular calcification by inhibiting Wnt5a signalling in vascular smooth muscle cells. Nat. Commun. 3:1077 doi: 10.1038/ncomms2087 (2012).